Mechanically selflocked chiral gemini-catenanes Mechanically interlocked and entangled molecular architectures represent one of the elaborate topological superstructures engineered at a molecular resolution. Here we report a methodology for fabricating mechanically selflocked molecules (MSMs) through highly efficient one-step amidation of a pseudorotaxane derived from dual functionalized pillar[5]arene (P[5]A) threaded by α,ω-diaminoalkane ( DA- n ; n =3–12). The monomeric and dimeric pseudo[1]catenanes thus obtained, which are inherently chiral due to the topology of P[5]A used, were isolated and fully characterized by NMR and circular dichroism spectroscopy, X-ray crystallography and DFT calculations. Of particular interest, the dimeric pseudo[1]catenane, named ‘gemini-catenane’, contained stereoisomeric meso-erythro and dl-threo isomers, in which two P[5]A moieties are threaded by two DA- n chains in topologically different patterns. This access to chiral pseudo[1]catenanes and gemini-catenanes will greatly promote the practical use of such sophisticated chiral architectures in supramolecular and materials science and technology. Since the pioneering work by Frisch and Wasserman on chemical topology [1] , mechanically interlocked and entangled molecular architectures have attracted much interest because of their fascinating topological features [2] , [3] as well as the increasing influences on materials science and nanotechnology [4] , [5] , [6] , [7] . Inspired partly by the mathematical, iconological and religious symbols, much progress has been made in the rational synthesis of the mechanically interlocked molecules (MIMs) with ever-growing complexity [8] , [9] , [10] , [11] , [12] , [13] , [14] . A vast variety of bi- and multi-component MIMs, including [ n ]rotaxanes ( n ≥2), [ n ]catenanes ( n ≥2) and [c n ]daisy chains ( n ≥2) [15] , [16] , [17] , [18] , have hitherto been synthesized. In contrast, the covalently linked single-component locked molecules, which may be called mechanically selflocked molecules (MSMs) [19] , have sporadically been reported. Typical examples of MSMs include pseudo[1]rotaxane [20] , [21] , [22] , pseudo[1]catenane [23] , [24] , pretzelane [25] , [26] , double-lasso rotamacrocycle [27] , [28] and molecular figure-of-eight [29] . Compared with the well-established MIMs, however, the construction of higher-order MSM systems still remains a challenge, mainly due to the lack of a convenient general synthetic route and the tremendous obstacles in both synthesis and characterization. 1-Hydroxybenzotriazole (HOBT), a widely used additive for peptide synthesis [30] , has also been applied to the synthesis of cyclic peptides [31] , [32] , which stimulated us to employ this reagent in the synthesis of pseudo[1]catenanes and single-component MSMs through amidation. In this study, we have applied HOBT to the synthesis of a series of MSMs and found that the amidation mediated by HOBT serves as the essential step for constructing these sophisticated topologies. Intriguingly, when a long α,ω-diaminoalkane was reacted with pillar[5]arene-dicarboxylic acid in the presence of a condensation reagent (EDCI) and HOBT, a new member of the MSM family was obtained and eventually identified as a dually threaded pseudo[1]catenane, or ‘gemini-catenane’ in addition to a singly threaded pseudo[1]catenane, both of which are conformationally stable and inherently chiral. Synthetic approach to MSMs The Pillar[5]arene (P[5]A) is a [1 5 ]paracyclophane derivative consisting of five 1,4-dialkoxybenzene units mutually connected at the 2- and 5-positions with a methylene bridge [33] . The circular oxygen alleys at the both portals of pillararene, analogous to crown ether, strongly bind dicationic organic and difunctional guests [34] , [35] , [36] , [37] . A1/A2-difunctionalized dimethylpillar[5]arene (DMP[5]A) [38] can be prepared by the partial oxidation of DMP[5]A [39] , [40] and subsequent modification. Exploiting these features of P[5]A, we designed A1/A2-dicarboxylato-DMP[5]A ( 4 ) as the wheel of pseudorotaxane and α,ω-diaminoalkane as the axle. As shown in Fig. 1b , 4 was prepared from 1,4-dimethoxypillar[4]arene[1]hydroquinone ( 3 ) in 81% yield through alkylation with ethyl bromoacetate and the subsequent hydrolysis. Dicarboxylic acid 4 was reacted with 1,8-diaminooctane ( DA-8 ) in the presence of 1-(3-dimethylaminopropyl)-3-ethylcarbodiimide hydrochloride (EDCI·HCl) (2.5 equiv.) and HOBT (2.5 equiv.) for 48 h in CHCl 3 at room temperature to afford 1a as a white solid (melting point: 290–292 °C) in 51% isolated yield. The chemical structure of 1a was fully characterized by 1 H NMR, 13 C NMR, IR and HRMS spectroscopies and also by X-ray crystallography. In the IR spectra, the C=O stretching vibration was shifted from 1,730 cm −1 in 4 to 1,681 cm −1 in 1a , indicating formation of the amide linkage (see Supplementary Figs 53 and 54 ). In the 1 H NMR spectra of 1a , the signals of axle methylene protons were greatly upfield-shifted to δ <0, as a consequence of the shielding effect of the pillararene’s aromatic rings (see Supplementary Fig. 5 ). The crystal structure of 1a ( Fig. 2a ) unambiguously revealed the formation of pseudo[1]catenane, in which the pillararene ring is threaded by the octamethylene chain. Since this pseudo[1]catenane is planar-chiral as is the case with pillar[5]arene, the enantiomer pair was resolved by chiral HPLC. The first and second fractions collected showed mirror-imaged circular dichroism (CD) spectra ( Supplementary Figs 68 and 69 ) and were assigned to ( pS )- and ( pR )- enantiomers of pseudo [1]catenane 1a , respectively, by comparison with the theoretical CD spectra of P[5]A simulated by using the density functional theory (DFT) [41] . 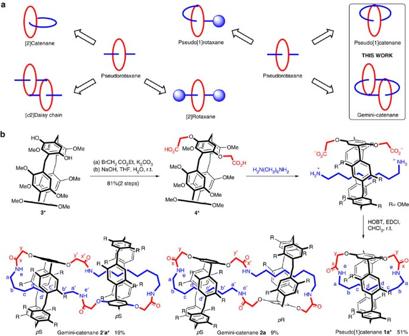Figure 1: Syntheses of pseudo[1]catenane and gemini-catenane. (a) MIMs and MSMs derived from pseudorotaxane. The original macrocyclic and acyclic components are indicated by red and blue colours, respectively. (b) Synthetic scheme of pseudo[1]catenane and gemini-catenane based on pillar[5]arene. *Only (pS)-enantiomers are shown for clarity purpose. Figure 1: Syntheses of pseudo[1]catenane and gemini-catenane. ( a ) MIMs and MSMs derived from pseudorotaxane. The original macrocyclic and acyclic components are indicated by red and blue colours, respectively. ( b ) Synthetic scheme of pseudo[1]catenane and gemini-catenane based on pillar[5]arene. *Only ( pS )-enantiomers are shown for clarity purpose. 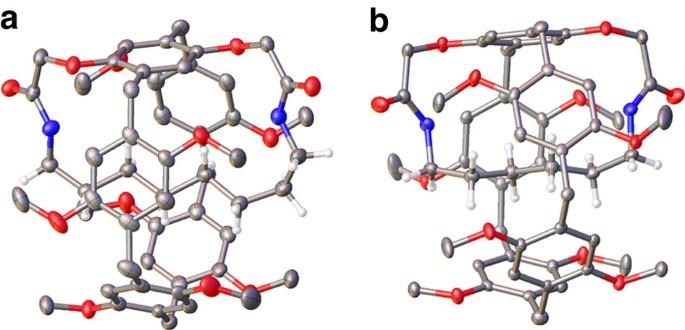Figure 2: Crystal structures of pseudo[1]catenanes. (a) Crystal structures of1a. (b) Crystal structures of1d. (Both of1aand1dthe thermal ellipsoids are at 50% probability). In the crystal structure, the hydrogen atoms of the pillararene moiety were omitted for clarity purpose; colour code: carbons in grey, hydrogens of the octamethylene moiety in white, oxygens in red and nitrogens in blue. Full size image Figure 2: Crystal structures of pseudo[1]catenanes. ( a ) Crystal structures of 1a . ( b ) Crystal structures of 1d . (Both of 1a and 1d the thermal ellipsoids are at 50% probability). In the crystal structure, the hydrogen atoms of the pillararene moiety were omitted for clarity purpose; colour code: carbons in grey, hydrogens of the octamethylene moiety in white, oxygens in red and nitrogens in blue. Full size image Interestingly, two additional products eluted by more polar solvents upon chromatographic separation were isolated in 9 and 19% yield, respectively. The HRMS analyses revealed their parent peaks in the ‘dimer’ region at m / z 1,894.9295 and 1,894.9445, respectively (see Supplementary Figs 46 and 47 ). Possessing exactly the twofold mass of 1a , these ‘dimeric’ products were assignable either to non-threaded 2:2 monocyclic dimers of 4 with DA-8 or to selflocked gemini-catenanes 2a and 2′a . The possibility of the non-threaded cyclodimers was immediately excluded on the basis of the unusually upfield-shifted octamethylene protons ( Supplementary Fig. 29 ). As a natural consequence of the planar chirality of pillararene [38] ( Fig. 1b ) and pre-assembled pseudorotaxane 4 used as a substrate in the present synthesis, the gemini-catenane generated therefrom should contain one S 2 -symmetric ‘erythro’ and two C 2 -symmetric ‘threo’ isomers. The catenane structure is obvious from the unusual upfield shifts of the octamethylene protons a−d in the 1 H NMR spectra ( Supplementary Fig. 29 ). More crucially, the two sets of protons a−d, which are equivalent to each other in 1a , are desymmetrized to give two significantly split series of protons a−d and a′−d′ in gemini-catenanes 2a and 2′a , revealing inequivalent magnetic environment for each series of the protons. Thus, the protons b−d are more deeply embedded into the pillararene cavity and suffer stronger shielding effects than the protons b′−d′ to show upfield shifts up to −1.97 p.p.m. in 2a and even to −2.33 p.p.m. in 2′a . The 13 C NMR spectra of 2a and 2′a confirm the above assignment. As can been seen from Fig. 3 , the carbonyl carbon (C x ) and the two methylene carbons (C a and C y ) adjacent to the amide group in 1a give single peaks, reflecting the equivalent magnetic environment for each of these carbons. In sharp contrast, all of the C a , C x and C y signals significantly split in both 2a and 2′a , indicating that the two amide groups are no longer equivalent in these molecules due to the gemini-catenane structure. 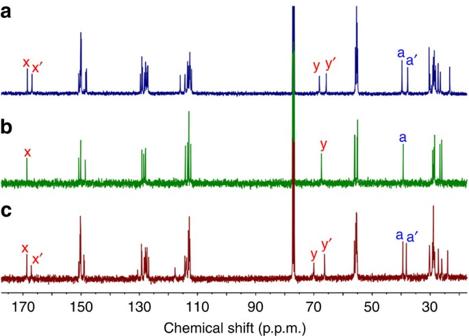Figure 3: Comparison of13C NMR spectra of MSMs. (a)13C NMR spectrum of2′a(100 MHz, CDCl3, 25 °C). (b)13C NMR spectrum of1a(100 MHz, CDCl3, 25 °C). (c)13C NMR spectrum of2a(100 MHz, CDCl3, 25 °C). The carbonyl (x) and adjacent methylene (a and y) carbons of pseudo[1]catenane1aare magnetically equivalent and show single peaks, while those of gemini-catenanes2aand2′asplit into two peaks, reflecting the inequivalent magnetic environment. Figure 3: Comparison of 13 C NMR spectra of MSMs. ( a ) 13 C NMR spectrum of 2′a (100 MHz, CDCl 3 , 25 °C). ( b ) 13 C NMR spectrum of 1a (100 MHz, CDCl 3 , 25 °C). ( c ) 13 C NMR spectrum of 2a (100 MHz, CDCl 3 , 25 °C). The carbonyl (x) and adjacent methylene (a and y) carbons of pseudo[1]catenane 1a are magnetically equivalent and show single peaks, while those of gemini-catenanes 2a and 2′a split into two peaks, reflecting the inequivalent magnetic environment. Full size image Chirality of gemini-catenanes The HRMS, 1 H NMR and 13 C NMR spectral analyses have unambiguously proven the gemini-catenane structure of 2a and 2′a , but did not allow us to discern these two stereoisomeric molecules. Nevertheless, their chiral structures and the relevant chiroptical properties enabled us not only to discern them but also to unequivocally assign their absolute configurations with the aid of circular dichroism (CD) spectra. From the symmetry point of view, gemini-catenane is either S 2 -symmetric (achiral) ‘erythro’ or C 2 -symmetric (chiral) ‘threo’, the former of which has a centre of symmetry and exists as a single meso-isomer, while the latter has no centre or plane of symmetry and therefore exists as a pair of enantiomers [42] , [43] , [44] . Knowing that, we performed the chiral HPLC analysis of these gemini-catenanes to find a single peak at 8.6 min for 2a but two well-separated peaks at 6.2 and 9.2 min for 2′a under the identical conditions (see Fig. 4a,b ), revealing that the former is achiral erythro and the latter chiral threo. 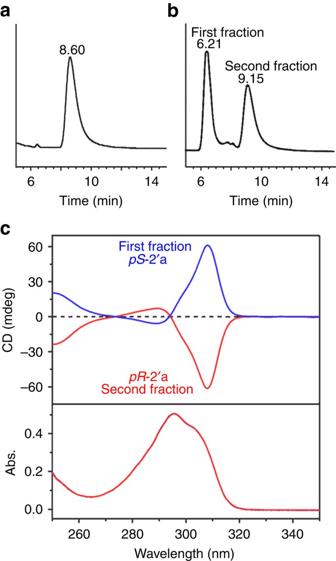Figure 4: Characterization of the chirality of gemini-catenane. (a) HPLC traces of2aon a chiral column. (b) HPLC traces of2′aon a chiral column. (c) UV/Vis and CD spectra of the first and second fractions. The existence of a single isomer in2aand a pair of enantiomers in2′awas confirmed by the chiral HPLC analyses and the mirror-imaged CD signals for the enantiomers of the latter ([pS-2′a]=[pR-2′a]=10 μM in CHCl3at 25 °C). Figure 4c illustrates the UV/Vis and CD spectra of the first and second fractions of 2′a , the absolute configurations of which were assigned to pS and pR , respectively, according to the same theoretical calculation of CD spectra of P[5]A [41] . Figure 4: Characterization of the chirality of gemini-catenane. ( a ) HPLC traces of 2a on a chiral column. ( b ) HPLC traces of 2′a on a chiral column. ( c ) UV/Vis and CD spectra of the first and second fractions. The existence of a single isomer in 2a and a pair of enantiomers in 2′a was confirmed by the chiral HPLC analyses and the mirror-imaged CD signals for the enantiomers of the latter ([ pS - 2′a ]=[ pR - 2′a ]=10 μM in CHCl 3 at 25 °C). Full size image Although all the attempts to crystallize the gemini-catenanes were unsuccessful, as shown in Fig. 5 , the DFT calculations revealed that 2a is more stable than 2′a by 0.8 kcal mol −1 . Interestingly, the Boltzmann distribution: 2′a : 2a= 3.7:1, evaluated by using the free energy difference, is close to relative isolated yield: 19%:9%=2.1:1 (see Supplementary Methods and references for computational details). 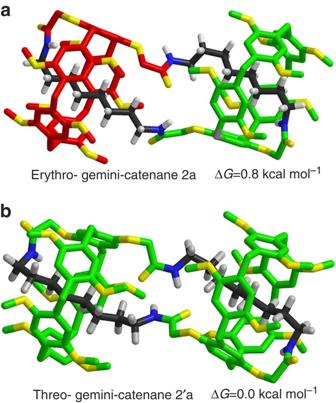Figure 5: Geometries and Gibbs free energies of gemini-catenanes2aand2′aoptimized by DFT calculations. The geometries were optimized by using the B3LYP/6-31G(d) method. M062X-D3 dispersion energy corrections are included in the reported Gibbs free energies. The Gibbs free energy of2ais given relative to2′a. Hydrogen atoms of pillararene components are omitted for clarity. The (pS)- and (pR)-pillar[5]arenes are shown in green and red, respectively. Figure 5: Geometries and Gibbs free energies of gemini-catenanes 2a and 2′a optimized by DFT calculations. The geometries were optimized by using the B3LYP/6-31G(d) method. M062X-D3 dispersion energy corrections are included in the reported Gibbs free energies. The Gibbs free energy of 2a is given relative to 2′a . Hydrogen atoms of pillararene components are omitted for clarity. The ( pS )- and ( pR )-pillar[5]arenes are shown in green and red, respectively. Full size image Robust conformation of MSMs In mechanically selflocked bicyclic structures, one of the incorporated macrocycles is often de-threaded from another macrocycle by aromatic ring tumbling [23] , [24] . If such de-threading took place in our molecules, the proton signals of the octamethylene chain would coalesce in 1 H NMR spectra. In our case, no essential chemical shift changes were observed for any of the proton signals of pseudo[1]catenane 1a in CDCl 3 even upon addition of an excess amount (10 equiv.) of competitor 1,4-dicyanobutane, which exhibits very strong binding affinities towards DMP[5]A [45] , and the octamethylene proton signals were consistently upfield-shifted even in more polar CD 2 Cl 2 , CD 3 CN and (CD 3 ) 2 SO, as shown in Supplementary Fig. 30 . We further performed the variable-temperature 1H NMR experiment in (CD 3 ) 2 SO to find no coalescence behaviour at least up to 80 °C. In addition, no new peaks (or products) were observed in the NMR spectrum of 1a even after heating at 160 °C for 2 h. Exactly the same experiments were repeated with gemini-catenanes 2a and 2′a to show no essential changes in the NMR spectra (see Supplementary Figs 32–37 ), indicating that the de-threading does not occur and hence 1a , 2a and 2′a are conformationally robust. Nevertheless, there still remains the possibility of de-threading by tumbling one of the aromatic rings under extreme conditions, and hence we may describe them as pseudo[1]catenanes or endo-spirocycles. Substrates scope with diaminoalkanes The scope and limitations of this facile route to MSMs were explored by employing DA- n of shorter and longer methylene chain lengths ( n =2–4, 6, 10 and 12). As shown in Table 1 , no catenanes were obtained in the reaction of DA-2 with 4 (entry g), most probably due to the dimethylene linker, which is too short to catenate at the both ends of 4 . Possessing a longer methylene chain, DA-3 , DA-4 and DA-6 (entries b−d) gave the corresponding pseudo[1]catenanes 1b , 1c and 1d in progressively increasing 60, 86 and 96% yield, but no gemini-catenanes were obtained. The almost quantitative yield of 1d may be attributed to the formation of highly stable pseudorotaxane DA-6 ⊂ 4 (with a 10 5 M −1 order affinity [46] ), which is driven by the appropriate linker length for catenating cyclization and the dual electrostatic interactions [47] of the dicationic axle (diammoniohexane [ DA-6 ·H 2 ] 2+ ) with the dianionic wheel (pillararene-dicarboxylate 4 2− ). However, such an ammonium-carboxylate pair is not favourable for amidation, because mechanistically the amidation pair should be charge-neutral. It is likely therefore that HOBT not only mediates the intermolecular amidation, but also stabilizes the guest in the pillararene cavity by forming a hydrogen-bond between the HOBT’s nitrogen and the amino hydrogen on DA-6 , as illustrated in Fig. 6 . This leads to the smooth catenating amidation in the pseudorotaxane in particular for DA-6 . Table 1 Synthesis of pseudo[1]catenanes 1 and gemini-catenanes 2 and 2′ through amidation of 4 with α,ω-diaminoalkanes DA- n in the presence of EDCI and HOBT*. 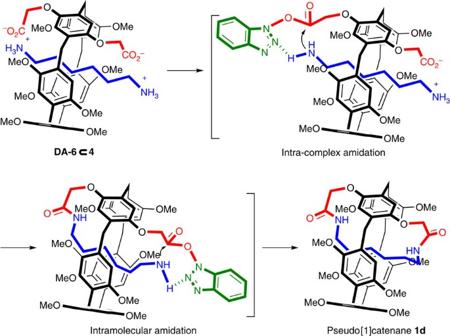Figure 6: A plausible reaction mechanism for the formation of1dmediated by HOBT. The amidation reaction can be promoted by the hydrogen-bonding interaction between HOBT and encapsulated diamine. Full size table Figure 6: A plausible reaction mechanism for the formation of 1d mediated by HOBT. The amidation reaction can be promoted by the hydrogen-bonding interaction between HOBT and encapsulated diamine. Full size image The use of longer diamine DA- n of n ≥8 led to the sudden formation of gemimi-catenanes 2 and 2′ at the expense of pseudo[1]catenane 1 ( Table 1 , entries a, e, f). With increasing methylene chain length ( n ), the yield of 1 markedly decreased from 96% at n =6 to 51% at n =8 and eventually to 23% at n =12. Interestingly, the combined yield of 2 and 2′ was kept constant at 28–29% over n =8–12 with an appreciable preference for chiral 2′ at smaller n . This unusual phenomenon can be rationalized with the help of the X-ray crystallographic structures of 1a and 1d ( Fig. 2a,b ). The pillararene cavity is perfectly fitted to the methylene chain length and the inter-amino distance of DA-6 , which leads to the almost quantitative yield of pseudo[1]catenane 1d . However, when a longer diamine ( n ≥8) is used, the first intra-complex amidation at one of the pillararene portals in the pseudorotaxane would proceed equally efficiently as shorter diamines, but the second intramolecular amidation at the other portal should be decelerated due to the longer distance between the coupling partners and the increased conformational flexibilities, which enhances the chance of intermolecular dimerization in gemini-catenane. Almost the same yields for gemini-catenanes of different chain lengths ( n =8–12) seem reasonable, because the chance of encounter would be comparable if the second intramolecular amidation is slow and the concentration of mono-amidated pre-pseudo[1]catenane is comparable for the longer diamines. Series of novel selflocked chiral pseudo[1]catenanes and gemini-catenanes were prepared in high yields in an HOBT-mediated one-pot synthesis starting from pillar[5]arene-dicarboxylic acid and α,ω-diamine substrates. The short diamines ( DA-3 , DA-4 and DA-6 ) exclusively afforded pseudo[1]catenanes in good to excellent yields. Crucially, the use of longer diamines ( DA-8 , DA-10 and DA-12 ) enabled us to obtain a new class of MSM, that is, gemini-catenane, as a consequence of the decelerated second catenating amidation of the conformationally more flexible [1]rotaxane intermediate precursor to pseudo[1]catenane. The gemini-catenane thus produced was a mixture of meso and dl diastereomers (due to the planar chirality of the pillararenes incorporated), which were successfully separated and clearly assigned to a single erythro and an enantiomer pair of threo isomers. The amidation mediated by HOBT is rather conventional but definitely essential to the formation of both pseudo[1]catenanes and gemini-catenanes, providing a convenient but powerful tool for synthesizing interlocked and selflocked molecules with well-defined structures. General 1,4-Dimethoxypillar[4]arene[1]hydroquinone (4DM1HQP5) [39] was synthesized according to the literature procedures. Solvents were used as received or dried according to the procedures described in the literature. TLC was performed on silica gel GF254 plates. Column chromatography was performed on silica gel (300–400 mesh). Melting points were measured on an RY-1A apparatus; the thermometer was not calibrated. 1 H NMR and 13 C NMR spectra were recorded on a Bruker AVANCE AV400 (400 and 100 MHz). Signal positions were reported in part per million (p.p.m.) relative to the residual solvent peaks or to the peak of Si(CH 3 ) 4 used as an internal standard with the abbreviations s, d, m, bs, and ABq, denoting singlet, doublet, multiplet, broad singlet and AB quartet, respectively. The residual 1 H peak of deuterated solvent appeared at 7.26 p.p.m. in CDCl 3 , at 5.32 p.p.m. in CD 2 Cl 2 , at 1.94 p.p.m. in CD 3 CN, and at 2.50 p.p.m. in (CD 3 ) 2 SO, while the 13 C peak of CDCl 3 at 77.0 p.p.m. All coupling constants J are quoted in Hz. FTIR spectra were obtained with a Bruker Tensor 27 instrument. All IR samples were prepared as thin film and reported in wavenumbers (cm −1 ). High resolution mass spectra (HRMS) were obtained on an Agilent 6520 Q-TOF LC/MS with ESI ionization. The X-ray diffraction data were collected by using a Rigaku Mercury CCD AFC10 system with monochromated Mo Kα radiation. Chiral HPLC analyses were performed on an Agilent 6890 Series instrument. The dimensions of the HPLC columns are 4.6 mm diameter, and 250 mm length. Circular dichroism (CD) spectra were recorded on a BioLogic MOS500 spectropolarimeter in a quartz cell of 10 mm light path. For 1 H and 13 C NMR spectra of compounds, see Supplementary Figs 1–28 . For the comparisons of 1 H NMR spectra of the 1a , 2a and 2′a , see Supplementary Fig. 29 . For the variable deuterated solvents and temperatures of 1 H NMR spectra of 1a , 2a and 2′a , see Supplementary Figs 30–37 . For HRMS spectra of compounds, see Supplementary Figs 38–51 . For IR spectra of compounds, see Supplementary Figs 52–65 . For the chiral HPLC traces and CD spectra of 1a and 2′a , see Supplementary Figs 68–74 . For crystallographic data of 1a and 1d , see Supplementary Table 1 . Synthetic procedures and spectroscopic and physical data of compounds see Supplementary Methods . For the DFT calculations of gemini-catenanes of 2a and 2′a , also see Supplementary Methods . For the Cartesian coordinates (Å), SCF energies and Gibbs free energies at 298 K for the optimized structures of 2a and 2′a , see Supplementary Data 1 . Syntheses of MSMs General procedures for the syntheses of pseudo[1]catenanes and gemini-catenanes: exemplified by the reaction of pillararene-dicarboxylic acid 4 with 1,8-diaminooctane DA-8 : HOBT (101 mg, 0.75 mmol) and EDCI (144 mg, 0.75 mmol) were added to a solution of 4 (251 mg, 0.30 mmol) and DA-8 (47 mg, 0.33 mmol) in chloroform (100 ml), and then the mixture was stirred for 48 h at room temperature. The reaction mixture was poured into 0.1 M aqueous HCl solution. The organic layer was washed with water, saturated aqueous NaHCO 3 solution and brine, dried over Na 2 SO 4 and concentrated. The residue was purified by column chromatography on silica gel eluted with CHCl 3 /MeOH of 200:1 to 50:1 ratio (v/v) to afford 1a as a white solid (120 mg, 51%): m.p. 290–292 °C; TLC (CHCl 3 :MeOH=30:1 v/v), R f =0.65; 1 H NMR (400 MHz, CDCl 3 ) δ 6.97 (s, 2H), 6.87 (s, 2H), 6.84 (s, 4H), 6.80 (s, 2H), 5.85 (bs, 2H), 4.68, 4.48 (ABq, 4H, J =16.4 Hz), 3.74–3.77 (m, 34H), 3.02 (bs, 2H), 2.80 (bs, 2H), 0.58–0.72 (m, 2H), 0.29–0.44 (m, 2H), −0.79 to −0.76 (m, 4H), −1.34 to −1.25 (m, 2H), −1.48 to −1.37 (m, 2H); 13 C NMR (100 MHz, CDCl 3 ) δ 168.7, 150.8, 150.2, 150.1, 148.6, 129.1, 128.5, 128.0, 127.9, 127.8, 114.2, 113.4, 113.0, 112.3, 67.4, 56.1, 55.9, 55.2, 55.0, 39.3, 29.2, 28.9, 28.7, 28.5, 26.7, 26.1; IR (KBr) ν max 3,415, 2,934, 2,853, 2,829, 1,681, 1,496, 1,464, 1,398, 1,212, 1,046, 928, 880, 856, 774, 727, 704, 646 cm −1 ; HRMS ( m / z ): [M+H] + calc. for C 55 H 67 N 2 O 12 , 947.4694; found, 947.4670. 2a , White solid (21 mg, 9%): m.p. 294–296 °C; TLC (CHCl 3 :MeOH=30:1 v/v): R f =0.57; 1 H NMR (400 MHz, CDCl 3 ) δ 6.86–6.97 (m, 20H), 6.73 (s, 2H), 5.08 (bs, 2H), 4.62, 4.55 (ABq, 4H, J =16.4 Hz), 4.47, 4.39 (ABq, 4H, J =16.4 Hz), 3.77–3.98 (m, 68H), 3.33 (bs, 2H), 3.23 (bs, 2H), 2.41 (bs, 2H), 1.69 (bs, 2H), 1.27 (bs, 4H), 0.62 (bs, 4H), −0.04 (bs, 4H), −1.01 (bs, 6H), −1.28 (bs, 2H), −1.97 (bs, 4H); 13 C NMR (100 MHz, CDCl 3 ) δ 168.7, 167.1, 150.9, 150.4, 150.2, 150.1, 149.1, 148.9, 130.6, 129.3, 129.1, 128.3, 128.2, 127.9, 127.7, 127.3, 126.8, 117.7, 114.4, 113.9, 113.7, 113.2, 112.9, 112.7, 112.6, 70.0, 66.3, 56.1, 55.6, 55.5, 55.4, 55.3, 55.2, 55.1, 39.4, 38.2, 30.4, 30.3, 30.2, 29.3, 29.0, 28.8, 28.7, 28.5, 27.2, 26.0, 24.0; IR (KBr) ν max 3,412, 2,933, 2,853, 2,829, 1,727, 1,680, 1,533, 1,498, 1,465, 1,399, 1,212, 1,047, 929, 880, 855, 774, 727, 704, 647 cm −1 ; HRMS ( m / z ): [M+H] + calc. for C 110 H 133 N 4 O 24 , 1,894.9343; found, 1,894.9295. 2′a , White solid (44 mg, 19%): m.p. 260–262 °C; TLC (CHCl 3 :MeOH=30:1 v/v): R f =0.52; 1 H NMR (400 MHz, CDCl 3 ) δ 6.84–7.05 (m, 20H), 6.84 (s, 2H), 5.23 (bs, 2H), 4.62 (s, 4H), 4.51 (s, 4H), 3.74–3.82 (m, 68H), 3.36 (bs, 4H), 2.67 (bs, 2H), 1.71 (bs, 2H), 1.47 (bs, 4H), 0.78 (bs, 4H), −0.08 (bs, 2H), −0.15 (bs, 2H), −1.09 (bs, 2H), −1.21 (bs, 2H), −1.45 (bs, 2H), −1.55 (bs, 2H), −2.33 (bs, 4H); 13 C NMR (100 MHz, CDCl 3 ) δ 168.5, 166.9, 150.8, 150.4, 150.2, 150.1, 150.1, 145.0, 148.4, 148.1, 129.6, 129.1, 128.9, 128.3, 127.9, 127.9, 127.7, 127.4, 127.2, 127.0, 115.9, 114.3, 113.4, 113.2, 112.8, 112.6, 112.5, 112.1, 68.1, 66.8, 55.7, 55.6, 55.4, 55.2, 55.1, 55.0, 39.7, 37.7, 30.4, 30.1, 29.1, 29.0, 28.7, 28.5, 28.2, 27.3, 26.6, 23.3; IR (KBr) ν max 3,411, 2,935, 2,854, 2,829, 1,680, 1,532, 1,498, 1,465, 1,398, 1,212, 1,046, 928, 880, 855, 774, 731, 704, 647 cm −1 ; HRMS ( m / z ): [M+H] + calc. for C 110 H 133 N 4 O 24 , 1,894.9343; found, 1,894.9445. Accession codes : For OLEX of products 1a and 1d , see Supplementary Figs 66 and 67. CCDC 1016257 and CCDC 1016258 contain supplementary crystallographic data for this paper. These data can be obtained free of charge from The Cambridge Crystallographic Data Centre via www.ccdc.cam.ac.uk/data_request/cif . How to cite this article: Li, S.-H. et al. Mechanically selflocked chiral gemini-catenanes. Nat. Commun. 6:7590 doi: 10.1038/ncomms8590 (2015).